New approach for rice improvement using a pleiotropic QTL gene for lodging resistance and yield The use of fertilizer results in tall rice plants that are susceptible to lodging and results in reduced plant yields. In this study, using chromosome segment substitution lines, we identified an effective quantitative trait loci (QTL) for culm strength, which was designated STRONG CULM2 ( SCM2 ). Positional cloning of the gene revealed that SCM2 was identical to ABERRANT PANICLE ORGANIZATION1 ( APO1 ), a gene previously reported to control panicle structure. A near-isogenic line carrying SCM2 showed enhanced culm strength and increased spikelet number because of the pleiotropic effects of the gene. Although SCM2 is a gain-of-function mutant of APO1 , it does not have the negative effects reported for APO1 overexpression mutants, such as decreased panicle number and abnormal spikelet morphology. The identification of lodging-resistance genes by QTL analysis combined with positional cloning is a useful approach for improving lodging resistance and overall productivity in rice. Food scarcity is becoming a serious global problem because of the constantly increasing world population and the effects of global climate change on food production [1] , [2] . In the 1960s, remarkable success was attained in increasing grain production through the development and widespread adoption of high-yielding, semidwarf varieties of wheat and rice. Extensive cultivation of these varieties led to a major increase in grain production, consequently averting a predicted large-scale famine. This phenomenal achievement was referred to as the Green Revolution [3] , [4] , [5] . A major factor in the Green Revolution was the widespread use of fertilizers in the cultivation of high-yielding, semidwarf varieties. Supplemental fertilization is not only essential for increasing grain yield, but also promotes stem and leaf elongation, resulting in an overall increase in plant height. Under heavy fertilization, traditional varieties of wheat and rice grow excessively tall and are susceptible to lodging, which breaks their basal culms and results in significant yield loss. In contrast, dwarf varieties respond to high fertilizer inputs and produce more grain because their short stature makes them resistant to lodging. Furthermore, semidwarf varieties have high tillering ability and harvest index. These are the major reasons why the Green Revolution doubled the yield in both wheat and rice [6] . The success of the Green Revolution convinced many breeders of the suitability of semidwarf varieties for increased crop productivity, and many improved semidwarf varieties have been developed and cultivated worldwide [7] , [8] , [9] . However, despite the short stature conferred by the semidwarf1 ( sd1 ) gene, lodging remains a problem in many of the improved rice varieties. In some wheat cultivars carrying the major dwarfing genes Rht1 and Rht2 , lodging was also observed [10] . Furthermore, heavy yield losses due to lodging have been observed in other crops [11] , [12] , [13] , [14] , [15] . In an effort to avert another looming food crisis, rice breeders are developing new varieties with increased plant biomass and harvest index to further increase the grain yield. Recently, several genes associated with grain yield have been identified, including GN1A [16] , GS3 [17] , DEP1 [18] and WFP [19] . However, to sustain this breeding objective, it is also necessary to develop new strategies to improve lodging resistance in rice. Instead of relying solely on the sd1 gene, major genes and quantitative trait loci (QTL) controlling culm strength can be used in developing improved rice varieties. However, genes associated with culm strength are yet to be identified and isolated. In this study, a QTL analysis combined with positional cloning led to the identification and isolation of a major QTL conferring lodging resistance in rice. A near-isogenic line (NIL) carrying this gene showed enhanced culm strength and increased spikelet number due to pleiotropic effects. These results suggest that breeding rice varieties with high grain yield and enhanced lodging resistance can now be approached using this pleiotropic QTL gene or other genes having similar functions. Culm morphology and lodging resistance in chromosome segment substitution lines To isolate genes conferring lodging resistance, the improved indica rice ( Oryza sativa ) variety, Habataki, was selected as the donor parent, as it produces very strong culms compared with the typical japonica varieties. Furthermore, chromosome segment substitution lines (CSSLs) from a cross between Habataki, and the japonica variety Sasanishiki (as the recurrent parent) is available [20] . Habataki produces about 300 grains per panicle, yet its plant architecture is capable of supporting heavy panicles ( Fig. 1a ). In fact, culm diameter and culm wall thickness of Habataki are much wider and thicker at the centre of internodes than that of japonica varieties such as Koshihikari and Sasanishiki ( Fig. 1b ). 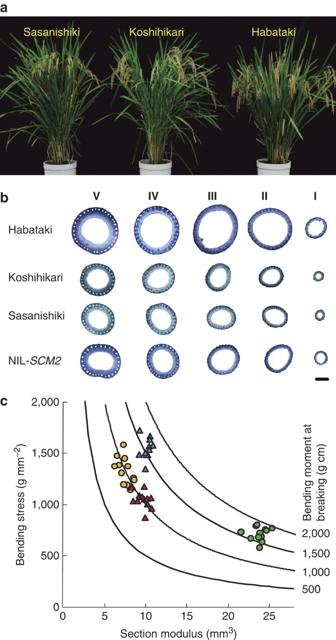Figure 1: Plant morphology and culm strength. (a) Plant morphology of Habataki andjaponicavarieties Sasanishiki and Koshihikari. (b) Cross-sections of the culm from the first internode (I: panicle-neck internode) to the fifth internode (V: basal internode). Scale bar: 2 mm. (c) Relationship between section modulus and bending stress. Curved lines indicate the bending moment of the fourth internode at breaking. Orange circle: Koshihikari, red triangle: Sasanishiki, blue triangle: NIL-SCM2, green circle: Habataki. Figure 1: Plant morphology and culm strength. ( a ) Plant morphology of Habataki and japonica varieties Sasanishiki and Koshihikari. ( b ) Cross-sections of the culm from the first internode (I: panicle-neck internode) to the fifth internode (V: basal internode). Scale bar: 2 mm. ( c ) Relationship between section modulus and bending stress. Curved lines indicate the bending moment of the fourth internode at breaking. Orange circle: Koshihikari, red triangle: Sasanishiki, blue triangle: NIL- SCM2 , green circle: Habataki. Full size image The bending moment at breaking (M), a parameter for the physical strength of the culm, was measured using the fourth internode of the plant. The M value of Habataki was much higher than that of Sasanishiki and Koshihikari ( Fig. 2 ). The M value can be further divided into two parameters: the section modulus (SM), which is directly influenced by the culm morphology (for example, diameter and wall thickness); and bending stress (BS), which is a function of culm cell wall components, such as cellulose and lignin. To determine the mechanism behind the high M value of Habataki, SM and BS were measured ( Figs 1c and 2 ). The SM of Habataki was over two times greater than that of the two japonica varieties. This very high SM value of Habataki can be attributed to its large and thick culm ( Fig. 1b ). On the other hand, the BS of Habataki was lower than that of the japonica varieties ( Figs 1c and 2 ), which indicates that the composition of the culm in Habataki is inferior to that in the japonica varieties with respect to lodging resistance. Actually, Sasanishiki, Koshihikari and most japonica varieties have high BS values because of elevated levels of lignin and cellulose in the culms [21] . These observations clearly indicate that lodging resistance in japonica varieties can be improved by incorporating the gene from Habataki that increases the culm diameter. 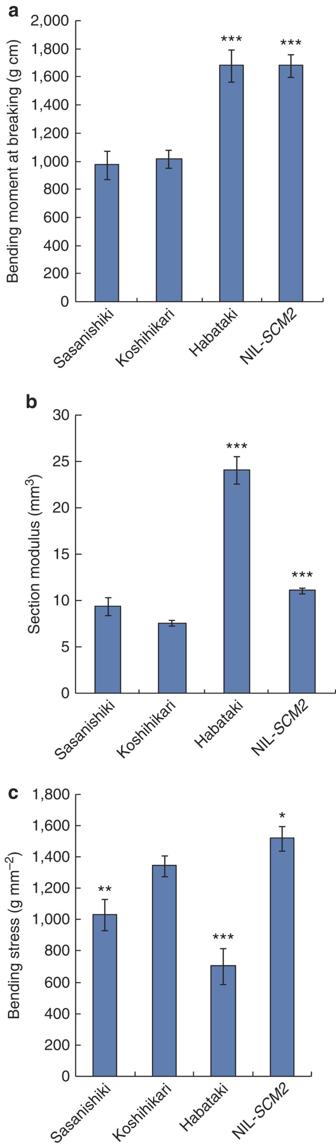Figure 2: Bending moment at breaking, section modulus and bending stress. (a) Comparison of the bending moment at breaking of the fourth internodes at 20 days after heading between Sasanishiki, Koshihikari, Habataki and NIL-SCM2. (b) The section modulus of the fourth internodes at 20 days after heading. (c) The bending stress of the fourth internodes at 20 days after heading. Each column represents mean±s.d. ***P<0.001, **P<0.01 and *P<0.05 versus Koshihikari (Dunnett's multiple comparison test, three replicates). Figure 2: Bending moment at breaking, section modulus and bending stress. ( a ) Comparison of the bending moment at breaking of the fourth internodes at 20 days after heading between Sasanishiki, Koshihikari, Habataki and NIL- SCM2 . ( b ) The section modulus of the fourth internodes at 20 days after heading. ( c ) The bending stress of the fourth internodes at 20 days after heading. Each column represents mean±s.d. *** P <0.001, ** P <0.01 and * P <0.05 versus Koshihikari (Dunnett's multiple comparison test, three replicates). Full size image To localize the loci responsible for high SM in Habataki, the M and SM values of the CSSLs were measured in 2005 and 2006 ( Fig. 3 ). Both parameters were clearly affected by the environment (growth conditions such as weather and soil), as most of the lines showed significantly higher values than the original variety (Sasanishiki) in 1 year but not the other year. However, two CSSLs (SL403 and SL420) showed significantly higher M and SM values than Sasanishiki in both years. Thus, the structure of the fourth internode of these lines was examined ( Supplementary Fig. S1 ). Compared with Sasanishiki, SL403 had thicker culm walls whereas SL420 had wider culm diameters. SL403 and SL420 carry a genome segment of chromosome (chr.) 1 and 6 from Habataki, respectively. Thus, the QTL located on Habataki chr. 1 is effective for increasing culm wall thickness, whereas the QTL on chr. 6 increases culm diameter. The QTL on chr. 1 and 6 were designated as STRONG CULM1 ( SCM1 ) and STRONG CULM2 ( SCM2 ), respectively. 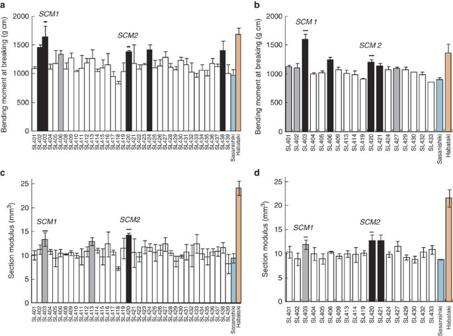Figure 3: Culm strength and culm thickness in CSSLs. (a) The bending moment at breaking of the fourth internodes at 20 days after heading in 2005. (b) The bending moment at breaking of the fourth internodes at 20 days after heading in 2006. (c) The section modulus of the fourth internodes at 20 days after heading in 2005. (d) The section modulus of the fourth internodes at 20 days after heading in 2006. Each column represents mean±s.d. Black bars: significant atP<0.001; grey bars: significant atP<0.01 versus Sasanishiki (Dunnett's multiple comparison test, three replicates). Blue bars: Sasanishiki (recurrent parent), orange bars: Habataki (donor parent). Figure 3: Culm strength and culm thickness in CSSLs. ( a ) The bending moment at breaking of the fourth internodes at 20 days after heading in 2005. ( b ) The bending moment at breaking of the fourth internodes at 20 days after heading in 2006. ( c ) The section modulus of the fourth internodes at 20 days after heading in 2005. ( d ) The section modulus of the fourth internodes at 20 days after heading in 2006. Each column represents mean±s.d. Black bars: significant at P <0.001; grey bars: significant at P <0.01 versus Sasanishiki (Dunnett's multiple comparison test, three replicates). Blue bars: Sasanishiki (recurrent parent), orange bars: Habataki (donor parent). Full size image Isolation and characterization of SCM2 For enhanced lodging resistance in japonica varieties, increasing the culm diameter is better than increasing the culm wall thickness. The SM of a hollow culm is calculated by a formulae that considers culm diameter ( d ) and culm wall thickness ( t ) [22] as follows: Apparently, culm diameter is more effective in increasing M and SM than the culm wall thickness, and requires less investment of biomass ( Supplementary Fig. S2 ). Thus, a wider culm diameter with a thinner culm wall maximizes lodging resistance without reducing yield potential. Hence, the isolation and further characterization of SCM2 was pursued instead of SCM1 . As the ultimate goal of this study is to utilize lodging-resistance genes in rice breeding programmes, a Koshihikari NIL with the introgressed SCM2 locus of Habataki was developed. Koshihikari has been the most popular variety in Japan for many decades, and lodging is the most serious problem in the cultivation of this variety. Using a BC 5 F 2 population generated from the cross between Koshihikari and its substitution line (SL) carrying the QTL SCM2 region in Habataki (15.8–124.4 cM of chr. 6), a segregation analysis for SM was conducted ( Fig. 4 ). The SM values of the segregating F 2 population ranged from 5.9 to 15.3 mm 3 . The SM distribution in Koshihikari homozygous, heterozygous and Habataki homozygous alleles was 5.9–10.9 mm 3 (mean of 7.6 mm 3 ), 7.4–15.3 mm 3 (mean of 11.2) and 7.5–14.9 mm 3 (mean of 12.1), respectively. These results indicate that the strong culm conferred by SCM2 is inherited in a semidominant manner. It also shows the obscure difference in the phenotype of plants representing the different genotypes, thus rendering the phenotyping of SCM2 a difficult and sensitive analysis. 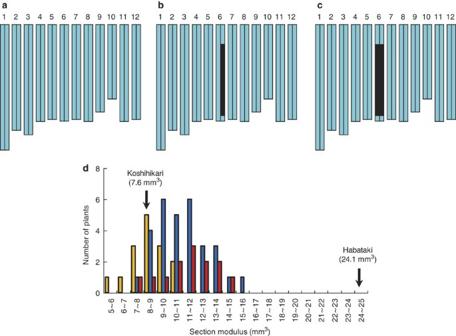Figure 4: Frequency distribution of section modulus in a BC5F2population. (a–c) Chromosome maps of Koshihikari (a), Koshi-QTLSCM2heterozygous (b) and Koshi-QTLSCM2homozygous (c). Black bars: 15.8–124.4 cM of the Habataki sixth chromosome. (d) Frequency distribution of the section modulus in a BC5F2population produced by crossing between Koshihikari and its substitution line carrying the QTLSCM2region (15.8–124.4 cM of the Habataki sixth chromosome). Orange, blue and red bars indicate the number of plants carrying the Koshihikari homozygous, Koshihikari heterozygous and Habataki homozygous allele at the QTLSCM2region (108.6 cM), respectively. Figure 4: Frequency distribution of section modulus in a BC 5 F 2 population. ( a – c ) Chromosome maps of Koshihikari ( a ), Koshi-QTL SCM2 heterozygous ( b ) and Koshi-QTL SCM2 homozygous ( c ). Black bars: 15.8–124.4 cM of the Habataki sixth chromosome. ( d ) Frequency distribution of the section modulus in a BC 5 F 2 population produced by crossing between Koshihikari and its substitution line carrying the QTL SCM2 region (15.8–124.4 cM of the Habataki sixth chromosome). Orange, blue and red bars indicate the number of plants carrying the Koshihikari homozygous, Koshihikari heterozygous and Habataki homozygous allele at the QTL SCM2 region (108.6 cM), respectively. Full size image A stepwise positional cloning of SCM2 ( Fig. 5a ) was performed for mapping experiments. For the precise phenotyping of SM, 20 SLs carrying homozygous alleles of the target region from 600 BC 5 F 3 plants were selected through marker-assisted selection (MAS). Each of these lines was phenotyped for the trait and compared with Koshihikari for two growing seasons. First, using the 20 SLs (BC 5 F 4 ), SCM2 was mapped to the long-arm region of chr. 6. After using 2,000 selfed progenies of heterozygous NIL- SCM2 for fine mapping, the candidate region was localized within 15 kb. In this region, there is only one gene, ABERRANT PANICLE ORGANIZATION1 ( APO1 ), which encodes an F-box-containing protein involved in controlling the rachis branch number of the panicle [23] . The sequences of APO1 in Koshihikari and Habataki were compared and were found to contain insertions, deletions, single-nucleotide polymorphisms and insertion of a large retrotransposon ( Fig. 5a ). Any of these variations may have caused the differences in APO1 function in the two varieties. 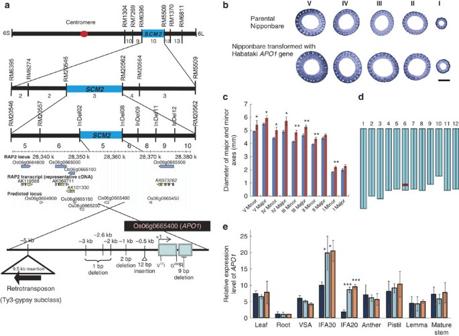Figure 5: Location and gene structure ofSCM2. (a) Location ofSCM2and comparison of the gene sequence ofAPO1between Habataki and Koshihikari. TheSCM2locus was predicted between the markers RM6395 and RM5509 on chromosome 6. Course mapping narrowed theSCM2locus between RM20546 and RM20562. The candidate region ofSCM2was narrowed down to the 15 kb between InDel02 and InDel08 by fine mapping. The number of recombinants between molecular markers is indicated below the maps. Nucleotide replacements are shown in Habataki against Koshihikari. (b) Culm cross-sections from the first (I: panicle-neck internode) to the fifth (V: basal internode) internodes in Nipponbare transformed with the HabatakiAPO1locus and an empty vector. Scale bar: 2 mm. (c) The diameter of major and minor axes from the first to the fifth internode of the main culms between theAPO1transgenic and control plants. Each column represents mean±s.d. (n=5); **P<0.01 and *P<0.05 (Student'st-test). (d) Graphical genotype of NIL-SCM2on rice chromosomes. The red bar indicates the chromosome segment (484 kb) of Habataki includingAPO1. (e) Expression analysis by real-time PCR ofAPO1in various organs. VSA, vegetative shoot apex, IFA30, inflorescence apex at 30 days before heading, IFA20, inflorescence apex at 20 days before heading. Each column represents mean±s.d. (three replicates); ***P<0.001; *P<0.05 versus Koshihikari (Dunnett's multiple comparison test). Figure 5: Location and gene structure of SCM2 . ( a ) Location of SCM2 and comparison of the gene sequence of APO1 between Habataki and Koshihikari. The SCM2 locus was predicted between the markers RM6395 and RM5509 on chromosome 6. Course mapping narrowed the SCM2 locus between RM20546 and RM20562. The candidate region of SCM2 was narrowed down to the 15 kb between InDel02 and InDel08 by fine mapping. The number of recombinants between molecular markers is indicated below the maps. Nucleotide replacements are shown in Habataki against Koshihikari. ( b ) Culm cross-sections from the first (I: panicle-neck internode) to the fifth (V: basal internode) internodes in Nipponbare transformed with the Habataki APO1 locus and an empty vector. Scale bar: 2 mm. ( c ) The diameter of major and minor axes from the first to the fifth internode of the main culms between the APO1 transgenic and control plants. Each column represents mean±s.d. ( n =5); ** P <0.01 and * P <0.05 (Student's t -test). ( d ) Graphical genotype of NIL- SCM2 on rice chromosomes. The red bar indicates the chromosome segment (484 kb) of Habataki including APO1 . ( e ) Expression analysis by real-time PCR of APO1 in various organs. VSA, vegetative shoot apex, IFA30, inflorescence apex at 30 days before heading, IFA20, inflorescence apex at 20 days before heading. Each column represents mean±s.d. (three replicates); *** P <0.001; * P <0.05 versus Koshihikari (Dunnett's multiple comparison test). Full size image To confirm that APO1 corresponds to SCM2 , a genomic DNA fragment containing the APO1 locus of Habataki was introduced into the japonica variety Nipponbare through Agrobacterium -mediated transformation. The APO1 transgenic plants showed a wider culm diameter at internodes as compared with the parental variety ( Fig. 5b,c ), indicating that APO1 regulates the diameter of culm internodes. Interestingly, the transgenic plants also showed a thicker culm wall than the parental variety Nipponbare ( Fig. 5b ), suggesting that SCM2 also regulates culm wall thickness, although no difference in culm wall thickness between SL420 and the original variety was observed ( Supplementary Fig. S1 ). On the basis of the observations of APO1 -overexpressing mutants [24] , different levels of APO1 expression had varying effects on the phenotype of plant organs, especially the rice panicle. As plants transformed with genomic DNA containing the APO1 locus may not be identical, the difference in phenotype between the introgressed and transgenic lines may be explained by differences in APO1 expression levels. Evaluation of SCM2 for lodging resistance To evaluate the effect of SCM2 on lodging resistance, an NIL carrying a 484-kb region from the distal part of chr. 6 of Habataki (NIL- SCM2 ; Fig. 5d ) was developed. There was no difference in the flowering time between NIL- SCM2 and Koshihikari. The APO1 expression levels in Koshihikari, NIL- SCM2 and Habataki were compared ( Fig. 5e ). The APO1 expression level in NIL- SCM2 was similar to Koshihikari in most of the plant organs. However, in the inflorescence apex at 30 and 20 days before heading, the APO1 expression level was about 2–3 times higher in NIL- SCM2 and Habataki as compared with Koshihikari. The culm diameter of NIL- SCM2 and Koshihikari was also compared. In NIL- SCM2 , the diameters of the minor and major axes in all the internodes were significantly wider than in Koshihikari ( Figs 1b and 6 ). Consequently, the SM of NIL- SCM2 was also higher than that of Koshihikari ( Fig. 2 ). The BS of Koshihikari and NIL- SCM2 was higher than that of Habataki ( Figs 1c and 2 ), but the M value of the NIL- SCM2 culm was sximilar to Habataki ( Fig. 2 ). The size of the inflorescence meristem of NIL- SCM2 was apparently larger than that of Koshihikari ( Fig. 7a,b ), and the number of parenchyma cells in the basal internode of NIL- SCM2 was about 38% higher than that in Koshihikari ( Fig. 7c–f ). These observations suggest that the high APO1 expression level in the inflorescence apex of NIL- SCM2 causes the increased culm diameter by promoting active cell division in the meristem (see Discussion ). 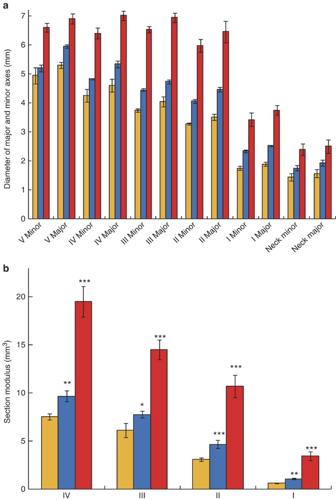Figure 6: Culm diameter and section modulus in NIL-SCM2in comparison with Koshihikari and Habataki. (a) Comparisons of diameter in major and minor axes from the neck node and the first (I: panicle-neck internode) to the fifth (V: basal internode) internodes among Koshihikari, NIL-SCM2and Habataki. Orange bars: Koshihikari, blue bars: NIL-SCM2, red bars: Habataki. Each column represents mean±s.d. (three replicates). (b) Comparisons of section modulus from the first to the fourth internodes among Koshihikari, NIL-SCM2and Habataki. Orange bars: Koshihikari, blue bars: NIL-SCM2, red bars: Habataki. Each column represents mean±s.d. (three replicates). ***P<0.001; **P<0.01; *P<0.05 versus Koshihikari (Dunnett's multiple comparison test). Figure 6: Culm diameter and section modulus in NIL- SCM2 in comparison with Koshihikari and Habataki. ( a ) Comparisons of diameter in major and minor axes from the neck node and the first (I: panicle-neck internode) to the fifth (V: basal internode) internodes among Koshihikari, NIL- SCM2 and Habataki. Orange bars: Koshihikari, blue bars: NIL- SCM2 , red bars: Habataki. Each column represents mean±s.d. (three replicates). ( b ) Comparisons of section modulus from the first to the fourth internodes among Koshihikari, NIL- SCM2 and Habataki. Orange bars: Koshihikari, blue bars: NIL- SCM2 , red bars: Habataki. Each column represents mean±s.d. (three replicates). *** P <0.001; ** P <0.01; * P <0.05 versus Koshihikari (Dunnett's multiple comparison test). 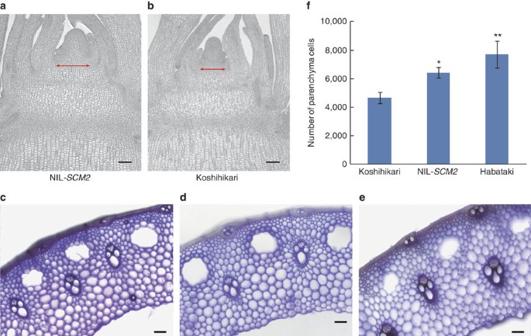Figure 7: Morphological characteristics of the shoot apex and the basal internode. (a,b) The longitudinal sections stained with propidiumiodide of the shoot apex region of Koshihikari (a) and NIL-SCM2(b) at 30 days before heading. The arrows indicate the diameter size at the basal part of panicle for each plant. Scale bar: 100 μm. (c–e) The cross-sections stained with crystal violet of the fourth internodes in Koshihikari (c), NIL-SCM2(d) and Habataki (e) at 20 days after heading. Scale bar: 100 μm. (f) The number of parenchyma cells in the cross-section area of the fourth internode of NIL-SCM2in comparison with Koshihikari and Habataki. Each column represents mean±s.d. (three replicates). **P<0.01; *P<0.05 versus Koshihikari (Dunnett's multiple comparison test). Full size image Figure 7: Morphological characteristics of the shoot apex and the basal internode. ( a , b ) The longitudinal sections stained with propidiumiodide of the shoot apex region of Koshihikari ( a ) and NIL- SCM2 ( b ) at 30 days before heading. The arrows indicate the diameter size at the basal part of panicle for each plant. Scale bar: 100 μm. ( c – e ) The cross-sections stained with crystal violet of the fourth internodes in Koshihikari ( c ), NIL- SCM2 ( d ) and Habataki ( e ) at 20 days after heading. Scale bar: 100 μm. ( f ) The number of parenchyma cells in the cross-section area of the fourth internode of NIL- SCM2 in comparison with Koshihikari and Habataki. Each column represents mean±s.d. (three replicates). ** P <0.01; * P <0.05 versus Koshihikari (Dunnett's multiple comparison test). Full size image To determine the usefulness of SCM2 in practical breeding, the performance of the gene was further evaluated under field conditions. 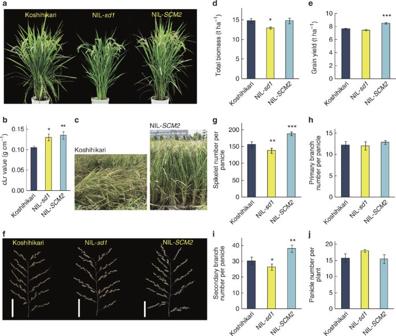Figure 8: Lodging resistance and yield performance of NIL-SCM2compared with Koshihikari and NIL-sd1. (a) Morphology of Koshihikari, NIL-sd1and NIL-SCM2at the ripening stage. (b) cLr values. (c) Comparison of lodging in Koshihikari and NIL-SCM2after a strong typhoon. (d,e) Comparison of total biomass production (d) and unhulled grain yield (e). (f) Panicle structure of Koshihikari, NIL-sd1and NIL-SCM2. Scale bars: 5 cm. (g–i) Comparison of spikelet (g), primary branch (h) and secondary branch (i) numbers per panicle observed from the main stem of Koshihikari, NIL-sd1and NIL-SCM2. (?j) Panicle number per plant among Koshihikari, NIL-sd1and NIL-SCM2. Each column represents mean±s.d. (three replicates). ***P<0.001; **P<0.01; *P<0.05 versus Koshihikari (Dunnett's multiple comparison test). Figure 8a shows the overall plant stature of Koshihikari, NIL- SCM2 and NIL- sd1 carrying the null allele of sd1 (ref. 16), which was widely used in the Green Revolution of rice [8] . NIL- SCM2 was similar in plant height to Koshihikari. On the other hand, NIL- sd1 was shorter because of a deficiency in gibberellin synthesis [8] , [25] . Apparently, the resistance of NIL- SCM2 against the bending type of lodging was improved. The measured value for the lodging-resistance factor (cLr) of the line showed that it was similar or slightly better than NIL- sd1 ( Fig. 8b ). Figure 8: Lodging resistance and yield performance of NIL- SCM2 compared with Koshihikari and NIL- sd1 . ( a ) Morphology of Koshihikari, NIL- sd1 and NIL- SCM2 at the ripening stage. ( b ) cLr values. ( c ) Comparison of lodging in Koshihikari and NIL- SCM2 after a strong typhoon. ( d , e ) Comparison of total biomass production ( d ) and unhulled grain yield ( e ). ( f ) Panicle structure of Koshihikari, NIL- sd1 and NIL- SCM2 . Scale bars: 5 cm. ( g – i ) Comparison of spikelet ( g ), primary branch ( h ) and secondary branch ( i ) numbers per panicle observed from the main stem of Koshihikari, NIL- sd1 and NIL- SCM2 . (? j ) Panicle number per plant among Koshihikari, NIL- sd1 and NIL- SCM2 . Each column represents mean±s.d. (three replicates). *** P <0.001; ** P <0.01; * P <0.05 versus Koshihikari (Dunnett's multiple comparison test). Full size image In the autumn of 2009, a typhoon hit the experimental field where Koshihikari and NIL- SCM2 were planted. Although there was severe lodging of plants in the Koshihikari plot, the NIL- SCM2 plants were not affected by the strong wind and remained standing ( Fig. 8c ). This unexpected observation strongly demonstrates the effectiveness of SCM2 in enhancing lodging resistance of a japonica variety. It also shows the potential of utilizing lodging-resistance gene(s) as a new approach in breeding rice varieties for improved lodging resistance. Effects of SCM2 on crop productivity Koshihikari, NIL- SCM2 and NIL- sd1 were also evaluated for the grain yield, and two important components of yield, the total biomass and spikelet number. The total biomass of NIL- SCM2 and Koshihikari was similar, whereas NIL- sd1 produced 87% less biomass than Koshihikari owing to its shorter height ( Fig. 8d ). More importantly, the grain yield per hectare of NIL- SCM2 was significantly higher than that of Koshihikari and NIL- sd1 ( Fig. 8e ). These differences in grain yield depend mainly on spikelet numbers; for example, NIL- SCM2 plants produced more spikelets per panicle than Koshihikari (for example, 188 per panicle for NIL- SCM2 as compared with 156 for Koshihikari; Fig. 8f,g ). Consequently, SCM2 increased the spikelet number of NIL- SCM2 by about 20%. This increase in spikelet number by SCM2 was caused mainly by the increase in the secondary branch number of the panicle ( Fig. 8h,i ). The secondary branch number per panicle of NIL- SCM2 was about 38, whereas Koshihikari had about 30 ( Fig. 8i ), resulting in an increase of 25%. The increase in the secondary branching of the panicle and spikelet number in NIL- SCM2 is a positive, pleiotropic effect of APO1 . Indeed, the transgenic plants carrying the Habataki APO1 gene showed a 20% increase in the spikelet number relative to the parental variety, Nipponbare ( Supplementary Fig. S3 ), although transgenic plants grown in the greenhouse produced fewer spikelets than plants grown in the field. In contrast to NIL- SCM2 , productivity of NIL- sd1 was considerably reduced in both total biomass and spikelet number ( Fig. 8d,g ). Previously, two papers reported an increased number of spikelets in APO1 -overexpressing mutants, apo1-D and Ur1 , but with a dramatic decrease in the panicle number per plant [24] , [26] . As this negative effect of APO1 on panicle number per plant decreases the crop productivity [26] , we compared the panicle number per plant of NIL- SCM2 and NIL- sd1 with Koshihikari ( Fig. 8j ). The panicle number per plant in NIL- SCM2 and Koshihikari was similar, whereas NIL- sd1 had slightly more panicles than Koshihikari, probably because of its short stature. Thus, in contrast to previously reported APO1 -overexpressing mutants, NIL- SCM2 shows a positive effect of APO1 , that is, an increase in the spikelet number per panicle without a decrease in the panicle number (see Discussion ). Therefore, SCM2 confers lodging resistance and also increases grain yield. To date, short plant stature has been the major target for improvement of lodging resistance in rice because it confers lower susceptibility to lodging and a higher harvest index. In fact, the use of semidwarf genes such as sd1 and Rht1 successfully eliminated the lodging problem in rice and wheat, respectively, and also increased the crop productivity [5] . However, in japonica varieties that normally produce weak and fine culms, sd1 is ineffective in enhancing the culm strength. Hence, the lodging resistance of these varieties has been improved by decreasing the length and weight of the above-ground parts of the plant [27] . The use of lodging-resistance genes in addition to the dwarfing gene is a promising new approach in improving lodging resistance and further increasing productivity in rice. Before this study, lodging-resistance genes had not been identified. It is possible that the genes involved in strong and/or thick culm also regulate the overall development of the culm, and often cause negative pleiotropic effects on the development of other organs, such as the leaf, flower and grain. Thus, we performed QTL analysis for lodging resistance using a high-yielding rice variety with strong, thick culms. From Habataki, an improved high-yielding indica variety with strong and thick culms, we isolated a QTL that effectively controls culm strength. This QTL, which was located on chr. 6 and designated as SCM2 , also increases the spikelet number of the panicle as a pleiotropic effect. Koshihikari NIL introgressed with SCM2 from Habataki showed significantly enhanced culm strength, increased spikelet number and grain yield. This result shows that the gene can be effective in improving lodging resistance, and yield in japonica varieties. It also indicates that the use of genes involved in culm strength can be used in breeding both japonica and indica varieties for increased lodging resistance. Although SCM2 is common among indica varieties, other QTL having similar action as SCM2 (for example, weaker alleles of Ur1 ) can be identified and used in indica breeding. Positional cloning and sequencing of SCM2 revealed that the gene is identical to APO1 , which encodes an F-box protein orthologous to Arabidopsis UFO [23] . Through detailed analysis of the APO1 -overexpressing mutant, apo1-D , Ikeda-Kawamitsu et al . [24] reported that APO1 regulates the cell proliferation rate in the inflorescence meristem. They further observed that a high expression level of APO1 increases the size of the inflorescence meristem, resulting in an increased number of spikelets. The isolation of apo1 -deficient mutants, which produce a smaller inflorescence meristem [23] , supports a positive role for APO1 in cell proliferation. Although previous studies on APO1 [24] , [26] , [28] focused on its effect on panicle structure, the increased cell division in the inflorescence meristem also impacts the size of the basal part of the inflorescence meristem ( Fig. 7a ); as a consequence, culm size is also affected because culm cells are produced from this region [29] . Thus, any increase in the cell proliferation rate in the inflorescence meristem inevitably leads to an increase in the spikelet number and culm diameter, both of which are favourable traits in terms of crop productivity. Why are overexpressing mutants of APO1 not used for practical breeding? Murai and Iizawa [30] observed an increased spikelet number in the APO1 -overexpressing mutant, Ur1 , and examined the possibility of mutating the gene to further increase the grain yield. According to their results, the number of spikelets per panicle of plants carrying homozygous or heterozygous Ur1 was about 200, which is 150% more than the original variety. However, the number of panicles per plant was reduced to about 75% in both genotypes; thus, the spikelet number did not differ significantly between the mutants and the wild variety. Moreover, the Ur1 plants exhibited decreased kernel weight and spikelet fertility and abnormal panicle morphology [31] , especially at lower temperatures [32] . The Hokkaido National Agricultural Experiment Station in Japan also attempted to develop high-yielding cultivars in its breeding program using the Ur1 mutant, but failed because of the abnormal phenotypes mentioned above. Similar undesirable but more severe abnormalities were observed in transgenic plants overproducing APO1 under the control of cauliflower mosaic virus 35S or maize UBIQUITIN promoter. These transgenic plants produced an excessively branched inflorescence without florets, and tiller outgrowth was suppressed [24] . Again, the severity of phenotype abnormalities exhibited by the plants was dependent on APO1- expression level, confirming that the APO1 affects the morphology of the panicle. When overexpressing mutants and NIL- SCM2 were compared, APO1 expression was higher in APO1- overexpressing mutants in various plant organs, including the inflorescence meristem. Whereas the expression level of the mutants was reportedly much higher than that of wild-type plants [24] , APO1 expression in NIL- SCM2 was only about two-fold higher than that in the parental variety ( Fig. 5e ). In the case of the Ur1 mutant, the increased level of expression of APO1 was observed in all parts of the seedlings 10 days after germination, whereas such upregulation was not observed in the vegetative tissues of NIL- SCM2 ( Fig. 5e ). The expression of APO1 in the vegetative tissues of the Ur1 mutant, therefore, may have caused the suppression of tiller outgrowth, resulting in a decreased panicle number per plant. Previously, we predicted possible situations in which conflicts between gene function and suitability of the trait affect the overall acceptability of an allele for breeding [33] . In this context, we discussed the possibility that alleles with greater gain-of-function may cause detrimental side effects to the trait that it is regulates. In such situations, an allele having a more moderate level of function is preferable to those with greatly increased function. For example, the APO1 alleles in the overexpressing mutants exhibit a large gain-of-function activity, with side effects not suitable for breeding. While these stronger alleles can significantly increase the spikelet number, they also reduce the panicle number per plant resulting in little or negative gain in grain yield. In contrast, the QTL SCM2 , a weaker allele of APO1 , is more suitable for breeding as it increases spikelet number without reducing panicle number. Identifying superior alleles of agriculturally important genes in natural variants can be accomplished through allele mining, an emerging new molecular approach in crop improvement. In the past, rice geneticists and breeders have collected and generated many rice mutant lines. However, most of these mutants have not been utilized in breeding programs because they convey undesirable or non-productive traits. However, the identification and proven effectiveness of SCM2 , a weak allele of APO1 , opens possibilities for finding superior and more suitable alleles in natural variants. Thus, a combination of mutant studies and QTL analysis using natural variation are important strategies for identifying genes that can further increase crop productivity. Plant cultivation for precise phenotyping Field experiments for the precise phenotyping of lodging-resistance traits were conducted at the Experimental Farm of Field Science Center, Tokyo University of Agriculture and Technology, in 2005–2009. Because the same cultivation practice was performed for all 5 years, only the cultivation methods for 2009 are described here. Seeds were sown in nursery boxes on 7 May 2009. Seedlings at the fifth-leaf stage were transplanted to a paddy field on Tama River alluvial soil using one seedling per hill on 28 May 2009. The planting density was 22.2 hills per m 2 , with a spacing of 15×30 cm. Manure was applied at the rate of about 20 tons per hectare before puddling, whereas complete fertilizer containing 14% each of N, P 2 O 5 and K 2 O was applied as a basal dressing at the rate of 50 kg N, P and K per hectare. The field was maintained under submerged conditions throughout the course of the experiments. The experiments were designed with three randomly arranged replicates (4 m 2 for each plot). Precise phenotyping for lodging-resistance traits The physical parameters of the main culm, which are closely associated with lodging resistance, were used for precise phenotyping. Eight main culms were sampled from each plot to determine the average leaf number, and the bending load at breaking was measured at a distance of 4 cm between two supporting points by the method of Ookawa and Ishihara [27] using a universal testing machine (Tensilon RTM-25, Orientec). The Tensilon is a useful tool for precise evaluation of lodging-resistance traits in rice. Physical parameters were calculated by the following formula [27] , [34] : . M is the bending moment of the basal internode at breaking (g cm). , where, a 1 is the outer diameter of the minor axis in an oval cross-section, b 1 is the outer diameter of the major axis in an oval cross-section, a 2 is the inner diameter of the minor axis in an oval cross-section and b 2 is the inner diameter of the major axis in an oval cross-section. BS is a mechanical parameter for lodging resistance, which is influenced by the chemical composition of the culm such as cellulose and lignin (see Results ). The lodging-resistance factor (cLr), a parameter for evaluating resistance to bending type of lodging was also measured. The cLr value of the plant was determined following the method of Grafius and Brown [35] . QTL detection using CSSLs Detection of QTL for lodging resistance was conducted in 2005 and 2006. A set of 39 CSSLs derived from the backcrossed progenies involving the japonica variety Sasanishiki (recurrent parent) and the high-yielding indica variety, Habataki [20] (donor parent), was used for the experiment. A QTL was considered to be present when the average value of three replicates was significantly different between a CSSL and the recurrent parent in 2 years, according to Dunnett's multiple comparison test. Mapping and NIL production with SCM2 To dissect the putative QTL for culm strength on chr. 6 of Habataki, a BC 5 F 2 population was generated from a cross between Koshihikari and its SL carrying the QTL SCM2 region. To map SCM2 , 20 plants with recombination in the vicinity of the QTL were identified from 600 BC 5 F 3 plants through MAS. Recombinant homozygous plants (BC 5 F 4 ) were then further selected from the selfed progenies of these 20 BC 5 F 3 plants on the basis of MAS and were used to further define the QTL region. The phenotype of the recombinant homozygous lines was compared with Koshihikari in 2008 and 2009. Similarly, NIL- SCM2 selected from the BC 5 F 3 generation using MAS was used to evaluate the effects of the QTL on lodging resistance for two consecutive seasons. Genomic DNA was extracted from leaves using the cethyltrimethylammonium bromide (CTAB) method [36] , and pure DNA samples were used for genotyping using single-sequence repeat markers [37] , [38] . Fine mapping and positional cloning of SCM2 A total of 2,000 selfed progenies (BC 5 F 3 ) of heterozygote NIL- SCM2 derived from the cross Koshihikari × Habataki were used for the combined analysis of fine mapping and positional cloning of SCM2 . Phenotyping of SCM2 was performed using the BC 5 F 5 generation. For fine mapping, single-sequence repeat markerss and newly developed InDel markers identified by using rice genome sequences in the NIAS and STAFF databases ( http://rgp.dna.affrc.go.jp ) were used. The primer sets of the InDel markers used are listed in Supplementary Table S1 . A Koshihikari BAC clone (J0018E09) covering the candidate region was selected from the BAC library and sequenced. DNA fragments of Habataki (HABA61H13) and Koshihikari within 10 kb of the candidate region were then compared. Transformation Full-length genomic DNA of APO1 , including the 5′ and 3′ regions (1.5 kb), was inserted to the binary vector pBI-Hm12, which contains a hygromycin-resistance gene. The DNA fragment was introduced into the japonica variety Nipponbare by Agrobacterium tumefaciens -mediated transformation. More than ten independent T 0 plants were generated and five plants were used for assay. As a control, transformants containing an empty vector were included, and used five control plants in each assay. RNA isolation and expression analysis Total RNA from various organs was prepared as described by Sambrook et al . [39] and was treated with DNase I. First-strand complementary DNA (cDNA) was synthesized from 1 μg of total RNA using an Omniscript reverse transcription kit (Qiagen). Quantitative real-time PCR was performed using the SYBR Green PCR Master Mix (Applied Biosystems) on an automated DNA sequence detector system (Model 7000; Applied Biosystems). The results were confirmed using three independent biological replicates. The UBC (AK059694; ubiquitin-conjugating enzyme E2) gene from rice was used as an internal standard for normalizing variations in cDNA concentration. The primer sets used for PCR are listed in Supplementary Table S2 . Observation for the longitudinal section of shoot apex Tissue samples were fixed overnight in 4% (v/v) paraformaldehyde in 25 mM NaPO 4 buffer, pH 7.0, at 4 °C. Samples were then dehydrated in a graded series of ethanol concentrations, infiltrated with the polymethacryl resin Technovit 7100 (Heraeus Kulzer), followed by embedding and polymerization in Technovit 7100, and were observed with a light microscope (BX-50; Olympus). Observation of the cross-section of basal internode The fourth internodes were sampled at 20 days after heading and fixed in FAA fix solution (formalin (35%): acetic acid: alcohol (70%) = 1:1:18). Tissue samples were stained by 0.05% crystal violet solution. The cross-section of internodes was observed with a digital microscope (SZX12; Olympus) and the parenchyma cells were counted using a digital image processing software (Win-ROOF version 6.0; Mitani). Statistical analysis Statistical comparison of multiple sets of data was carried out using Dunnett's multiple comparison test and Tukey's significant difference test. How to cite this article: Ookawa, T. et al . New approach for rice improvement using a pleiotropic QTL gene for lodging resistance and yield. Nat. Commun. 1:132 doi: 10.1038/ncomms1132 (2010).